Source identification of the Arctic sea ice proxy IP25 Analysis of the organic geochemical biomarker IP 25 in marine sediments is an established method for carrying out palaeo sea ice reconstructions for the Arctic. Such reconstructions cover timescales from decades back to the early Pleistocene, and are critical for understanding past climate conditions on Earth and for informing climate prediction models. Key attributes of IP 25 include its strict association with Arctic sea ice together with its ubiquity and stability in underlying marine sediments; however, the sources of IP 25 have remained undetermined. Here we report the identification of IP 25 in three (or four) relatively minor (<5%) sea ice diatoms isolated from mixed assemblages collected from the Canadian Arctic. In contrast, IP 25 was absent in the dominant taxa. Chemical and taxonomical investigations suggest that the IP 25 -containing taxa represent the majority of producers and are distributed pan-Arctic, thus establishing the widespread applicability of the IP 25 proxy for palaeo Arctic sea ice reconstruction. The reconstruction of sea ice conditions in the polar regions represents a key objective within palaeoceanography and palaeoclimatology [1] . This is largely owing to the major role that sea ice has in controlling the energy budget at the Earth’s surface, due to its high albedo, and also since it limits heat, gas and moisture exchange between the oceans and the atmosphere [2] , [3] . Further, sea ice contributes to ocean ventilation and circulation via brine rejection and freshwater input, following formation and melting, respectively [2] . Performing such reconstructions is challenging, however, since sea ice itself leaves no direct legacy signature in geological archives, necessitating the use of so-called proxy methods. A number of proxies for sea ice exist and these are both biogenic [1] and non-biogenic in origin [4] , [5] , [6] . Within the former category, the recent discovery of the organic geochemical biomarker IP 25 (ref. 7 ) (a C 25 highly branched isoprenoid (HBI) lipid [8] ) has attracted considerable interest, not least because it possesses the unique attribute of being produced within the sea ice itself. Consistent with this sea ice origin, the occurrence of IP 25 in marine sediments shows a strong correlation, spatially, to seasonally ice-covered Arctic waters [9] , and, from a temporal perspective, IP 25 appears to be stable in sediments for millions of years [10] . Combined, these attributes of IP 25 have provided the foundation for decadal to millennial-scale sea ice reconstructions across the Arctic [9] , [10] , [11] , [12] , [13] , [14] , [15] . Despite these interesting and valuable applications of the IP 25 sea ice proxy, the source organisms responsible for formation of this lipid in sea ice have remained elusive. A diatom source has been proposed [7] , [16] , however, since IP 25 has been reported in Arctic sea ice biota dominated by diatoms [16] , [17] and similar lipids occur in some non-sea ice algae [18] , [19] , [20] , [21] , [22] . More specifically, it has been hypothesized that sea ice diatoms belonging to the Haslea genus are likely producers of IP 25 on the basis of biosynthesis of related biomarkers by such species [7] , [16] , [17] , [23] , [24] , [25] . Nevertheless, IP 25 has never been reported in any cultures of diatoms, including some Haslea species isolated from Arctic sea ice [9] . Arguably, until the sources of IP 25 have been determined, together with information regarding their distributions across the Arctic, the potential for IP 25 as a palaeo sea ice proxy cannot be fully realized. In the current study, we identify three (or four) sea ice endemic diatom species that are responsible for IP 25 production in Canadian Arctic sea ice during a spring bloom. We achieve this by isolation of individual cells from mixed sea ice diatom assemblages and analysis of their lipid composition by gas chromatography–mass spectrometry (GC–MS). The identified IP 25 producers ( Pleurosigma stuxbergii var. rhomboides (Cleve in Cleve and Grunow) Cleve, Haslea kjellmanii (Cleve) Simonsen, H. crucigeroides (Hustedt) Simonsen and/or H. spicula (Hickie) Lange-Bertalot) constitute a relatively minor proportion of the ice taxa, but, significantly, they are nonetheless common pan-Arctic species that validate the notion that IP 25 represents a widespread proxy for palaeo Arctic sea ice. Identification of IP 25 producers Taxonomic assessment of the diatom assemblage within several algal aggregates from Resolute Bay in the Canadian Arctic revealed a distinctive flora, characteristic of sea ice [26] , [27] , [28] . Thus, the three most abundant species were Navicula pelagica ( ca . 40–50%), Nitzschia frigida ( ca . 10–20%) and Pauliella taeniata ( ca . 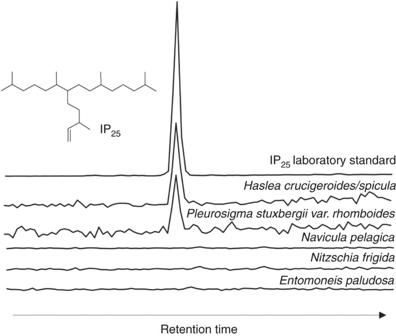Figure 1: Lipid extracts from isolated diatoms. Structure of IP25and partial GC–MS (selective ion monitoring;m/z350.3) chromatograms of lipid extracts obtained from various diatoms isolated from the mixed assemblages together with that of an authentic sample of IP25(ref.57). 10–20%) ( Table 1 ), with a near absence of planktic cells (<0.5%). From one assemblage (SIA-1), we isolated and combined sufficient numbers of cells from (at least) six individual species to perform quantitative lipid analysis by GC–MS to show that IP 25 was present in P. stuxbergii var. rhomboides and at least two species from the genus Haslea ( H. kjellmanii , H. crucigeroides and/or H. spicula ) ( Fig. 1 ), but was absent in other important ice algal species; N. pelagica , N. frigida , and Entomoneis paludosa ( Fig. 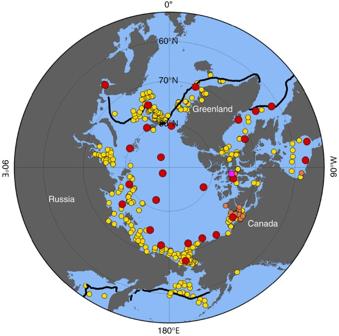Figure 2: Distribution of IP25producers and presence of IP25in sediments. Summary map showing locations where IP25has been identified in Arctic surface sediments (yellow circles) and sea ice (orange circles) (Supplementary Data 1). Red circles indicate the approximate locations of sea ice taxonomic studies reportingHasleaspp. andPleurosigma stuxbergii var. rhomboides(summarized inTable 1). The pink square shows the collection location of the ice algal aggregates analyzed in the current study. The black line shows the median March sea ice extent (National Snow and Ice Data Center; 1981–2010). 1 and Table 2 ). Table 1 Taxonomic composition of diatom aggregates. Full size table Figure 1: Lipid extracts from isolated diatoms. Structure of IP 25 and partial GC–MS (selective ion monitoring; m/z 350.3) chromatograms of lipid extracts obtained from various diatoms isolated from the mixed assemblages together with that of an authentic sample of IP 25 (ref. 57 ). Full size image Table 2 HBI content of isolated cells. Full size table The occurrence of IP 25 in H. crucigeroides (and/or H. spicula ) and H. kjellmanii is consistent with the production of other HBIs by members of the genus Haslea [18] , [19] , [25] , [29] , [30] , [31] , which led to the previous suggestion that Haslea was a likely source of IP 25 in Arctic sea ice [7] , [16] , [23] , [24] , despite the failure for such species to produce IP 25 in culture [29] . The identification of P. stuxbergii var. rhomboides as an IP 25 producer is also consistent with the formation of other HBIs by several Pleurosigma diatoms [20] , [32] , although we are unaware of any reports describing the HBI content of P. stuxbergii var. rhomboides , per se . In contrast, IP 25 was absent in at least two of the typically abundant ice flora ( viz, N. pelagica and N. frigida ), supporting the notion that IP 25 is produced selectively by a limited number of Arctic sea ice diatom taxa [7] , [16] , [23] , [24] . Indeed, the same conclusion was reached following taxonomic analysis and lipid characterization of mixed diatom assemblages in sectioned sea ice cores collected from the same location as the samples described here [16] . Previously, it has been shown that, although the physiology of diatom genera can be important for production of HBIs, not all species within such genera are HBI producers. Thus, some species within the Haslea , Pleurosigma and Navicula genera are known HBI producers, but others are not. For example, species such as H. ostrearia [18] and P. intermedium [32] produce HBIs, but H. wawrikae and P. angulatum do not [29] . Within the current context, we note that IP 25 was identified in H. kjellmanii , but was absent in H. vitrea ( Table 2 ). IP 25 was also found in H. crucigeroides and/or H. spicula ; however, since H. crucigeroides and/or H. spicula could not be distinguished during the cell isolation (see Methods section), we are unable to conclude whether both (or only one) of these are IP 25 producers. IP 25 and other HBIs were absent in cells of N. pelagica ( Table 2 ), despite the production of HBIs by some species of Navicula [22] . The absence of IP 25 in N. frigida is not surprising, however, since there have been no reports of HBI production in the genus Nitzschia . In addition to IP 25 , the structurally related di-unsaturated HBI biomarker C 25:2 [9] was also identified in each of the IP 25 -producing species ( Table 2 ). Previous studies based on the analysis of IP 25 in sea ice and sediments have shown a consistent abundance relationship between these two structural homologues indicating a common source at least within the Arctic [12] , [24] , [33] , [34] . Our data not only confirm this source association but, the similarity of the C 25:2 /IP 25 ratio in producers (2.3±0.8) to that found in sea ice and sediments [12] , [24] , [33] , [34] , implies a close link between the source and Arctic sedimentary signatures of these two biomarkers. As such, a significant formation of IP 25 over C 25:2 (or vice versa ) in sea ice or differential degradation of either biomarker in situ , seems unlikely. Finally, the ranges of intracellular concentrations of IP 25 and C 25:2 in the isolated sea ice diatoms were similar between individual species ( Table 2 ) and to those of HBIs measured in culture [16] . Major IP 25 -producing taxa The species selected for lipid analysis corresponded to ~65% of the total taxa in SIA-1, with IP 25 producers representing only 1.8% of the total. As such, the absence of IP 25 in the abundant N. pelagica and N. frigida corresponded to ~63% of total cell numbers. Although not all species were investigated (mainly because of low cell numbers of many minor species), these data suggest that the majority of sea ice diatom cells do not synthesize IP 25 ( Tables 2 and 3 ), which is consistent with previous lipid-based estimates that indicated only the minority of sea ice flora (1–5%) likely contribute to IP 25 biosynthesis [7] , [16] . Of course, it remains feasible that some other minor taxa may also be IP 25 producers but, given the low percentages of all unexamined species, together with the consistency in cellular abundances of those taxa that are producers, we suggest that their contributions are not significant. In support of this, we note that none of the unexamined genera ( Table 1 ) are known HBI producers. 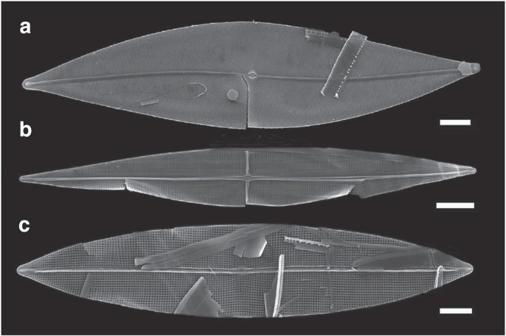Figure 3: IP25-producing diatom species. Scanning electron micrographs of IP25-producing diatoms identified in SIA-1. (a)Pleurosigma stuxbergii var. rhomboides; (b)Haslea crucigeroides(and/orHaslea spicula); and (c)Haslea kjellmanii. Scale bars, 10 μm. Table 3 Reported presence of IP 25 -producing diatoms in sea ice and IP 25 in Arctic sediments. Full size table In order to confirm that H. crucigeroides (and/or H. spicula ), H. kjellmanii and P. stuxbergii var. rhomboides indeed represented the majority (at least) of the IP 25 -producing species, and that the unanalyzed cells were not significant contributors to the IP 25 budget, we calculated the HBI abundance of SIA-1 relative to the total organic carbon (TOC) content (HBI/TOC=0.05%) and compared this ratio with the corresponding value obtained from a previously known HBI-producing species ( H. ostrearia ) in culture (HBI/TOC=1.4%). The ~30 times lower contribution of HBIs to sea ice algal TOC compared with that found for cultured diatoms provides a reasonable estimate of the percentage of HBI-producing diatoms in the sea ice algal assemblage (~3.6%). This low percentage confirms the relatively small proportion of IP 25 producers in the total assemblage, while the close similarity of this estimate to the combined percentages of H. crucigeroides (and/or H. spicula ), H. kjellmanii and P. stuxbergii var. rhomboides between SIA-1–4 ( Table 2 ) indicates that these species represent the majority (if not all) of the IP 25 producers. Having identified the major contributors of IP 25 in sea ice from a single study location in the Canadian Arctic, we next aimed to address the significance of this discovery with respect to the wider scale applicability of the IP 25 biomarker for palaeo sea ice studies. To do this, we compiled literature accounts of P. stuxbergii var. rhomboides, H. kjellmanii, H. crucigeroides and H. spicula (note: the latter two as separate species), and compared findings with reports of IP 25 in sediments (and sea ice). A summary of the spatial relationship between the two is shown in Fig. 2 . Figure 2: Distribution of IP 25 producers and presence of IP 25 in sediments. Summary map showing locations where IP 25 has been identified in Arctic surface sediments (yellow circles) and sea ice (orange circles) ( Supplementary Data 1 ). Red circles indicate the approximate locations of sea ice taxonomic studies reporting Haslea spp. and Pleurosigma stuxbergii var. rhomboides (summarized in Table 1 ). The pink square shows the collection location of the ice algal aggregates analyzed in the current study. The black line shows the median March sea ice extent (National Snow and Ice Data Center; 1981–2010). Full size image According to Poulin [35] , Haslea and Pleurosigma are typical of sea ice biota with five common taxa between them. H. crucigeroides , H. kjellmanii and H. spicula are identified as Arctic/sub-Arctic in distribution [35] , while H. crucigeroides and P. stuxbergii var. rhomboides are the most commonly reported ( Table 1 ). Owing to the close similarity between H. crucigeroides and H. spicula [36] , their occurrences may have been combined in some investigations, as has been the case here for the cell isolation and extraction experiments (see Methods section). Despite their widespread occurrence, however, H. crucigeroides, H. kjellmanii, H. spicula and P. stuxbergii var. rhomboides are always relatively minor taxa, with abundances usually <5% ( Table 3 ), as we found here ( Table 1 ). Individual studies have reported these IP 25 -producing species in first-year sea ice for locations ranging from 58 to 87 o N, including coastal, shelf and deep ocean environments. Further, such species have been reported in sea ice of varying thickness (for example, 4–300 cm) [37] , [38] and type [28] , [39] . With respect to biomarker-based studies, IP 25 has also been reported in surface and downcore sediments from across the Arctic, as reviewed by Belt and Müller [9] , while here, we demonstrate the excellent spatial relationship between occurrences of IP 25 in Arctic surface sediments (and sea ice) and reports of the IP 25 -producing diatoms identified in the current study ( Table 3 and Fig. 2 ). For example, H. crucigeroides, H. kjellmanii, H. spicula and P. stuxbergii var. rhomboides have been identified in sea ice from across the Canadian Arctic and sub-Arctic ( Table 1 ), and IP 25 has been identified as a common component in surface sediments from these regions, with downcore abundances providing the basis for Holocene sea ice reconstructions [9] , [13] , [40] , [41] . Similarly, in the eastern Arctic, where H. crucigeroides, H. kjellmanii, H. spicula and P. stuxbergii var. rhomboides are also common, IP 25 occurrence in recent sediments from the Kara, Laptev and Barents Sea shows a strong correlation with modern sea ice cover [24] , [42] , and this has aided the reconstruction of Holocene (and older) sea ice records from these regions [10] , [43] . Further, the observation of IP 25 -producing diatoms in sea ice from around Svalbard and the North East Polynya (NE Greenland) is consistent with the occurrence of IP 25 in nearby surface sediments [42] , [44] , and the longest IP 25 -based palaeo sea ice records to date are also from this region [10] , [45] . The majority of these IP 25 studies have been conducted in relatively shallow marine settings, proximal to continental shelves while, in contrast, there is currently a paucity of data from deeper oceanographic settings such as the Greenland Sea or the central Arctic Ocean. For the latter, in particular, it has been suggested previously that the combined presence of thick multi-year ice, likely unsuitable for diatom growth, and low sediment accumulation rates may somewhat limit the application of the IP 25 proxy method for palaeo sea ice reconstruction [9] . However, within the context of recent climate change and a reduction in both Arctic sea ice extent and thickness [46] , [47] , in particular, multi-year ice is becoming increasingly replaced by thinner first-year ice [48] . Consistent with such a change, we note that some of the IP 25 producers identified here have, in fact, been reported in first-year ice within the central Arctic (87 o N) [49] , and IP 25 has recently been detected in surface sediments >80 o N (X. Xiao and R. Stein, personal communication). We suggest that such observations, in combination with our results here, will likely expand the potential for the IP 25 proxy to provide palaeo sea ice reconstruction data for the entire Arctic. Previously, the identification of IP 25 in Arctic sediments has been interpreted as proxy evidence for past seasonal sea ice cover, with variations in sedimentary abundance attributed to corresponding changes in sea ice; an approach supported by a number of meaningful reconstructions [9] . In contrast, the possible influence of ecological controls over IP 25 production and their potential impact on its sedimentary abundance have been largely ignored, although its likely importance has been alluded to [7] , [9] , [16] . Having now identified those species that are responsible for IP 25 formation, it should be possible, in the future, to not only discuss ecological factors when interpreting sedimentary IP 25 distributions, but also to test the significance of these experimentally, and in an informed manner. Here, we suggest that the relatively consistent contribution of IP 25 producers to mixed Arctic sea ice diatom assemblages ( Table 3 ) provides some evidence that the larger temporal changes in IP 25 concentration often seen in sediments [9] , [12] , [13] , [40] , [45] are more likely attributable to sea ice variations than major modifications to diatom assemblage composition, although changes in overall production may still be important. On the other hand, relatively small or subtle variations in sedimentary abundance may, potentially, simply reflect minor changes in species composition or overall production rather than variations in sea ice cover. What is now clear, however, is that since IP 25 production is species specific and restricted to the minority diatom taxa, conclusions from future investigations into environmental or phenotypic variables over IP 25 production will require investigations of specific species, probably via in situ measurements in the field, rather than whole assemblage or simple biomass determinations. In this respect, the discovery of the IP 25 producers represents a key step in determining the factors that control the production and fate of IP 25 , which have been identified as important for its development as a palaeo sea ice proxy [9] . Sample collection Four floating ice algal aggregates (SIA-1–4) were collected from a sampling hole cut in first-year ice at Resolute Bay in association with the Arctic-ICE (Ice Covered Ecosystems) project (1–9 June 2012; 74 o 43.613′N; 95 o 33.496′W; Fig. 2 ). Aggregates consisted of sea ice algal assemblages recently sloughed from the underside interstitial channels of first-year ice and were stored in Whirl-Pak bags and frozen (−20 °C). A taxonomic description of the content of sectioned ice cores collected from the same location is given elsewhere [16] . Species identification Taxonomic identification of diatom species was carried out on each aggregate ( Table 1 ). Sub-samples of each of SIA-1–4 were freeze-dried, and ~10 mg of dried material was re-suspended in 100 ml of artificial seawater. Aliquots (0.5 ml) were taken for cell enumeration using the Utermöhl method [50] . Cell counts (400–600) were performed on parallel transects using an inverted microscope (Nikon Ti-S) at × 60 magnification [51] , [52] . More detailed examination of certain taxa was achieved by dry-mounting sub-samples of cleaned (10% HCl; 70 °C for 30 min and 3 × 10 ml Milli-Q washes) cells and examination using a JEOL 7001 F scanning electron microscope. Specifically, diatoms belonging to the genus Haslea ( Fig. 3 ) were identified based upon general morphological dimensions in addition to features considered characteristic of the genus including, for example, the presence of external longitudinal strips over many areolae, with intervening continuous slits [35] , [53] , [54] . Additional characteristic features included elongated helictoglossae, a well-defined accessory rib on the primary side of the raphe sternum and typically straight external raphe fissures with only slight terminal deflection/expansion [53] . Although both H. crucigeroides and H. spicula were identified in the assemblages as part of the detailed taxonomic analysis (Tatarek, Poland), it was not possible to distinguish between these two species during the low magnification (× 40) cell isolation stage (Brown, UK) because of the close similarities between them [36] . For P. stuxbergii var. rhomboides , identification was confirmed from the characteristic sigmoidal valve displaying fine striae, with slightly denser oblique than transverse pattern [55] and equally thickened primary and secondary raphe sternum ( cf . Gyrosigma [54] ; Fig. 3 ). Figure 3: IP 25 -producing diatom species. Scanning electron micrographs of IP 25 -producing diatoms identified in SIA-1. ( a ) Pleurosigma stuxbergii var. rhomboides ; ( b ) Haslea crucigeroides (and/or Haslea spicula ); and ( c ) Haslea kjellmanii . Scale bars, 10 μm. Full size image Total organic carbon Sub-samples (~50 mg) of freeze-dried algae were decarbonated (10% HCl; 10 ml), washed (3 × 10 ml Milli-Q water) and freeze-dried (−80°C; 0.001 mbar; 24 h) before analysis using a Thermoquest EA1110 CHN analyser. L -cystine was used as a calibration standard. Extraction and analysis of lipids Lipids were extracted from bulk algal aggregates and combined cells of individual species. For analysis of bulk aggregates, ~50 mg of each aggregate was first washed (3 × 10 ml Milli-Q water) to remove marine salts before being freeze-dried (−80 °C; 0.001 mbar; 24 h) and re-weighed before extraction. For extractions of individual diatom species, non-washed aggregate sub-samples were re-suspended in ~3 ml filtered (0.2 μm) artificial seawater (deionized water; 32 p.p.t. Tropic Marin salt) in a clean glass Petri dish. Individual diatom cells were identified using a Nikon TS2000 inverted light microscope (× 10 and × 40 objectives) in phase contrast and isolated manually using a modified Pasteur pipette. Following addition of an internal standard (9-octylheptadec-8-ene; 2 μg), bulk aggregates were saponified (20% KOH; 80 °C; 60 min) and extracted with hexane according to Brown et al . [17] , whereas for isolated cells a total hexane extract only was obtained (hexane; 3 × 1 ml, ultrasonication; 3 × 5 min). In each case, the resulting total hexane extract suspensions were filtered through pre-extracted (dichloromethane/methanol) cotton wool to remove cells before being partially dried (N 2 stream) and fractionated into non-polar lipids by column chromatography (hexane (3 ml)/SiO 2 ). Analysis of partially purified non-polar lipids was carried out using GC–MS techniques [56] with minor modifications to increase instrument sensitivity. Identification of IP 25 was achieved by a characteristic mass spectral response ( m/z 350.3; Fig. 1 ) using selective ion monitoring and co-injection of extracts with an authentic standard of IP 25 (ref. 57 ). Quantification was achieved by integrating the m/z 350.3 ion responses of IP 25 and the internal standard in selective ion monitoring mode, and normalizing the ratio between them using an instrumental response factor [56] and the number of cells extracted. How to cite this article: Brown, T. A. et al . Source identification of the Arctic sea ice proxy IP 25 . Nat. Commun. 5:4197 doi: 10.1038/ncomms5197 (2014).